A sensitive two-photon probe to selectively detect monoamine oxidase B activity in Parkinson’s disease models The unusually high MAO-B activity consistently observed in Parkinson’s disease (PD) patients has been proposed as a biomarker; however, this has not been realized due to the lack of probes suitable for MAO-B-specific detection in live cells/tissues. Here we report the first two-photon, small molecule fluorogenic probe (U1) that enables highly sensitive/specific and real-time imaging of endogenous MAO-B activities across biological samples. We also used U1 to confirm the reported inverse relationship between parkin and MAO-B in PD models. With no apparent toxicity, U1 may be used to monitor MAO-B activities in small animals during disease development. In clinical samples, we find elevated MAO-B activities only in B lymphocytes (not in fibroblasts), hinting that MAO-B activity in peripheral blood cells might be an accessible biomarker for rapid detection of PD. Our results provide important starting points for using small molecule imaging techniques to explore MAO-B at the organism level. Monoamine oxidases (MAOs) are mitochondria-bound flavoenzymes that catalyse the oxidative deamination of biogenic and dietary amines to their corresponding aldehydes, with the production of hydrogen peroxide (H 2 O 2 ) and ammonia in the process [1] . Two isoforms—that is, MAO-A and -B—are highly expressed in the human brain and have been differentiated based on their cellular/tissue localization, substrate preference, inhibitor sensitivity and physiological roles they play [2] , [3] , [4] . MAO-A is mainly localized in catecholaminergic neurons, metabolizes several different neurotransmitters and is selectively inhibited by clorgyline. MAO-B, on the other hand, is primarily found in astrocytes (and in some cases serotonergic neurons), acts on dopamine (DA) and β-phenylethylamine and is selectively inhibited by pargyline/rasagiline/L-deprenyl (selegiline). Together, these two enzymes assist in maintaining the homoeostasis of neurotransmitters in the brain, thereby ensuring appropriate neurological and behavioural outcomes [2] . Overactivation of these enzymes has been shown to cause excessive production of neurotoxic byproducts (for example, H 2 O 2 ), thus promoting neuronal dysfunctions that give rise to both psychiatric disorders and neurodegenerative diseases [5] , [6] . Take Parkinson’s disease (PD) for example, which is more common in older people. It has been shown that the expression of MAO-B, but not MAO-A, increases with age and its activity is significantly enhanced in the brain of PD patients [2] , [7] , [8] . The main pathology of PD is the loss of dopaminergic neurons near the substantia nigra pars compacta (SNpc) of the midbrain, a region populated with a high number of MAO-B-expressing astrocytes [9] . Under normal conditions, DA homoeostasis in these neurons is properly maintained by MAO-A-mediated breakdown of post-synaptic DA following its reuptake, as well as by the scavenging actions of neighbouring astrocytes that metabolize the internalized neurotransmitter via the action of MAO-B [2] , [10] . In PD patients, the elevation in MAO-B activity causes highly membrane-permeable H 2 O 2 generated to diffuse from astrocytes to neighbouring neuronal cells, which consequently leads to oxidative stress and their eventual degeneration. Notably, both selegiline and rasagiline are FDA-approved drugs for the treatment of early-stage PD, and they work by selectively inhibiting overexpressed MAO-B activity in the patients [11] , [12] , [13] . MAO-A-selective inhibitors such as clorgyline, however, are devoid of such therapeutic effects. In order to better understand the critical role that MAO-B plays in brain disorders and physiological consequences of its selective inhibition, especially for PD patients, technologies capable of sensitive and continuous monitoring of MAO-B activity in complex biological systems (that is, live cells, deep tissues and insects/animals) are urgently needed. Of the various types of standard assays employed to detect MAO activities [14] , [15] , [16] , [17] , [18] , [19] , [20] , [21] , [22] , advanced fluorescence-based methods might be suitable in this context [23] , owing to their practicality, high sensitivity and amenability to deep-tissue bioimaging (that is, by using near-infrared [24] or two-photon techniques [25] ); however, few provide any MAO-A/B selectivity [22] . For example, the commercially available Amplex Red kit and ELISA kit (ab109912), as well as several other existing fluorimetric approaches [14] , [15] , [16] , measures the fluorescent product liberated from the oxidation of the corresponding amine substrate by MAOs, in many cases with the assistance of a secondary enzyme or activating reagent (for example, NaIO 4 ). Chang and co-workers [19] reported a small molecule resorufin-based probe capable of live-cell imaging of MAO activities. Other studies based on similar design principles but with different fluorogenic MAO substrates have also been reported [18] , [20] . Recently, Ahn and co-workers [21] described the first two-photon MAO probe based on a dye called IminoPOS. None of these methods, however, confer any kind of selectivity in distinguishing the two MAO isoforms and thus is not suitable for above-mentioned applications. Previous attempts in the design of a MAO-B-specific fluorogenic probe based on an α-carbon oxidation mechanism catalysed by the enzyme on a MAO-B-specific substrate, 4-phenoxy-1-methyl-1,2,3,6-tetrahydropyridine were met with limited success [22] . While the resulting small molecule probe worked well for selective detection of recombinant MAO-B activity in vitro , it is not compatible for live-cell and other in vivo applications. Here we report the first two-photon, small molecule enzymatic probe, named U1 , which enables highly sensitive, specific and real-time imaging of MAO-B activities in various types of biological samples. Of the nine different probes designed and synthesized, we first establish the enzyme–probe interactions by using in silico docking experiments. We next investigate their photochemical, photophysical and enzymatic properties and subsequently confirm that U1 was indeed a highly selective probe to monitor MAO-B activities in recombinant proteins and mammalian lysates. Two-photon imaging experiments using mouse brains illustrate the ability of U1 to report endogenous MAO-B activity in deep tissues. Additional work with a series of well-established PD models (for example, from insects to human-derived samples) further highlights the utility of U1 for the sensitive detection of aberrant MAO-B expression during pathological development. Finally, U1 -based measurements of MAO-B status in human B lymphocytes validate the potential clinical values of U1 for analysis of disease progression in PD patients, opening up future prospects for non-invasive imaging-based diagnostic applications [26] , [27] . Design principle of the MAO probes In order to couple MAO-B-specific detection with high-resolution, real-time imaging in deep tissues such as the 200-μm-thick Drosophila brain (an established PD model [28] ), we turned to two-photon fluorescence microscopy, which, in addition to deep penetration (up to 1 mm in depth), offers several other advantages over one-photon fluorescence microscopy, including higher resolution, lower tissue autofluorescence and self-absorption, and reduced photodamage and photo-bleaching [25] , [29] . A number of small molecule two-photon probes have so far been developed to detect different biological targets [29] , [30] ; however, few can image enzymatic activities in live cells and deep tissues [21] , [31] , [32] , [33] , [34] , [35] . Probes capable of two-photon imaging of MAO-B-specific activities in live cells and tissues are at present not available. The most important feature in our probe design is therefore the MAO-B-specific fluorescence ‘Switch-ON’ behaviour. On the basis of the reported literature [22] , as well as in silico docking results ( vide infra ), we hypothesized that MAO-B-specific probes might be attainable by fine-tuning the MAO-reactive propylamine group and the two-photon fluorescence reporter, which were in turn linked by a self-immolative carbamate moiety ( Fig. 1 ). We chose 2-methylamino-6-acetylnaphthalene (acedan) and the conjugated pyrimidine derivative shown in Fig. 1c as the fluorogenic reporters due to their different molecular sizes and excellent properties in live-cell/tissue imaging [29] , [34] . We further introduced N -monomethylation and N , N -dimethylation to the propylamine group, as alkylated states of propylamine were previously shown to respond differentially to MAOs [17] , [18] , [19] , [20] . In total, nine probes, including the acedan-based (U1/2/3; Fig. 1b ) as well as both the asymmetric (U4/5/6) and symmetrical pyrimidine derivatives (U7/8/9; Fig. 1c ), were synthesized for the present study. 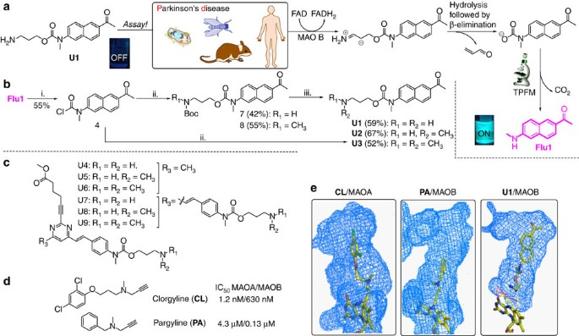Figure 1: Overview of the design and synthesis of potential MAO-B-specific probes. (a) Overall MAO-B-specific detection strategy by usingU1as a representative example. The method is used for fluorescence detection and (one- and two-photon) bioimaging of MAO-B activitiesin vitro, in live mammalian cells, Drosophila, mice and B lymphocytes isolated from PD patients. (b) Chemical synthesis ofU1/2/3: (i) trichloromethyl chloroformate, pyridine/dichloromethane (DCM) at 0 °C, room temperature for 12 h; (ii)tert-Boc-3-hydroxypropylamine/tert-Boc(3-hydroxypropyl)methylamine/3-dimethylamino-1-propanol for 7/8/U3, respectively, TEA/DCM at 0 °C, RT for 6 h; (iii) trifluoroacetic acid/DCM at 0 °C, RT for 3 h. (c) Chemical structures ofU4–9. SeeSupplementary Methodsfor synthesis. (d) Structure of irreversible MAO-A-seletive inhibitor clorgyline (CL) and MAO-B-selective inhibitor pargyline (PA). (e) Docked structures of CL/MAO-A, PA/MAO-B andU1/MAO-B, with only the surface of the active-site cavity shown in ‘chicken-wire’ representations (blue) and the compound shown in stick drawings. For other docked structures, seeSupplementary Fig. 1. Figure 1a summarizes the overall MAO-B detection strategy, by using U1 as a representative example. Initially U1 is in an ‘OFF’ state in which the intrinsic fluorescence of acedan is significantly quenched by the neighbouring electron-poor carbamate bond. Upon MAO-B-catalysed oxidation of the amino group to aldehyde (through an imine intermediate), a propionaldehyde moiety is released spontaneously by β-elimination followed by self-immolative discharge of CO 2 to liberate the electron-rich, highly fluorescent acedan (also labelled as Flu1 in the scheme). Here the utilized mechanism is an enzyme-induced process that causes both blockage of the photoinduced electron transfer (PeT) process and changes in the intramolecular charge transfer state of the reporter dye [36] . Similarly, the pyrimidine-based probes (for example, U4 –9), if processed enzymatically, would eventually liberate the highly fluorescent Flu2 and Flu3 as well ( Supplementary Methods ). Figure 1: Overview of the design and synthesis of potential MAO-B-specific probes. ( a ) Overall MAO-B-specific detection strategy by using U1 as a representative example. The method is used for fluorescence detection and (one- and two-photon) bioimaging of MAO-B activities in vitro , in live mammalian cells , Drosophila , mice and B lymphocytes isolated from PD patients. ( b ) Chemical synthesis of U1 /2/3: (i) trichloromethyl chloroformate, pyridine/dichloromethane (DCM) at 0 °C, room temperature for 12 h; (ii) tert -Boc-3-hydroxypropylamine/ tert -Boc(3-hydroxypropyl)methylamine/3-dimethylamino-1-propanol for 7/8/U3, respectively, TEA/DCM at 0 °C, RT for 6 h; (iii) trifluoroacetic acid/DCM at 0 °C, RT for 3 h. ( c ) Chemical structures of U4 –9. See Supplementary Methods for synthesis. ( d ) Structure of irreversible MAO-A-seletive inhibitor clorgyline (CL) and MAO-B-selective inhibitor pargyline (PA). ( e ) Docked structures of CL/MAO-A, PA/MAO-B and U1 /MAO-B, with only the surface of the active-site cavity shown in ‘chicken-wire’ representations (blue) and the compound shown in stick drawings. For other docked structures, see Supplementary Fig. 1 . Full size image On the basis of our design principle, as a representative, the synthetic scheme of U1 /2/3 is shown in Fig. 1b . U4 –9 were similarly synthesized ( Supplementary Methods ) [29] , [35] , [37] . Docking experiments were carried out to delineate the binding preference of our newly designed probes towards human MAO-A and -B ( Fig. 1d,e ). The binding of two isoform-specific inhibitors, clorgyline (CL) and pargyline (PA) against MAO-A and -B, respectively, was used as a reference ( Fig. 1e ); in spite of high structural similarity in the two isozymes, there are significant differences in their actives sites [38] . In the case of MAO-A, its active site contains a single hydrophobic cavity of 550 Å 3 (ref. 39 ). In contrast, the MAO-B active site is longer and narrower and consists of an ‘entrance’ cavity (290 Å 3 ) and a hydrophobic ‘substrate’ cavity (490 Å 3 ) occupied by the redox-active isoalloxazine ring of FAD coenzyme at the distal end [2] , [39] . Four residues (Tyr326, Ile199, Leu171 and Phe168) form the boundary between these two cavities and, upon binding, the inhibitor must negotiate through a loop (residues 99–112). Subsequent docking experiments were carried out with U1 /4/7, and the results indicate that these probes bound to MAO-B in distinctly different manners. In the case of U4 /7, both probes appeared to bind only to the surface of the protein, indicating that these probes might be too large to fit into the enzyme active site ( Supplementary Fig. 1 ). On the contrary, U1 fitted snugly into the ‘substrate’ cavity of MAO-B (Tyr60, Gln65, Val82, Glu84, Leu88, Leu171, Cys172, Ile198, Ile199, Ser200, Thr201, Glu207, Thr314, Ile316, Tyr326, Leu328, Met341, Phe343, Tyr398 and Tyr435) [39] , with its primary amine positioning towards the FAD coenzyme in close proximity (4.1 Å between the amine nitrogen in U1 and C5 in FAD; see Fig. 1e and Supplementary Fig. 2 ). Conversely in the U1 /MAO-A structure, the same amine was shown to point in the opposite direction and away from the ‘substrate’ cavity of the enzyme (Tyr69, Gln74, Val91, Val93, Leu97, Ile180, Asn181, Ile207, Phe208, Ser209, Val210, Glu216, Cys323, Ile325, Ile335, Leu337, Met350, Phe352, Tyr407 and Tyr444; Supplementary Fig. 2 ). These docking results thus provide the first line of evidence that U1 (and probably U2 /3 as well) could act as a MAO-B-specific probe. In support of this, similar docking experiments were performed with tyramine, a substrate recognized by both enzymes ( Supplementary Fig. 2 ); results showed that, unlike U1 , tyramine bound to both MAO-A and MAO-B in a similar orientation, with its primary amine pointing towards the FAD ring (3.6 and 5.7 Å between the amine nitrogen in tyramine and C5 in FAD for MAO-A and MAO-B, respectively). Chemical and biological properties of U1 and related probes To unequivocally establish that U1 indeed is a highly specific MAO-B imaging probe suitable for real-time live-cell and deep-tissue experiments, we first investigated its photophysical, photochemical and enzymatic properties ( Table 1 ). For comparison, other probes were concurrently tested ( Supplementary Table 1 and Supplementary Figs 3–7 ); under physiological conditions (HEPES buffer supplemented with 0.1% Triton X-100 at pH=7.5), all the primary, secondary and tertiary probes containing the same reporter dye exhibited almost identical absorption and emission behaviours—for example, U1 /2/3, U4 /5/6 and U7 /8/9 had absorption/emission maxima at 305/450 nm ( ε 305 =21,000 M −1 cm −1 , Φ =~0.10), 325/479 nm ( ε 325 =40,000 M −1 cm −1 , Φ <0.01) and 355/539 nm ( ε 355 =50,000 M −1 cm −1 , Φ =0.24), respectively. Interestingly, the parental reporters (Flu1, Flu2 and Flu3) showed red-shifted absorption/emission maxima at 352/498 nm ( ε 352 =24,000 M −1 cm −1 , Φ =0.19), 384/511 nm ( ε 384 =15,000 M −1 cm −1 , Φ =0.15) and 441/543 nm ( ε 441 =37,000 M −1 cm −1 , Φ =0.31), respectively. This is likely due to a greater delocalization of the lone-pair electrons in the methylamine group of the reporter, which is electron-donating and would stabilize the dye’s excited state [36] . The presence of an electron-poor carbamate bond, however, would reduce this effect in the probe. Additionally, the significantly brighter one- and two-photon excited fluorescence emission in Flu1 ( ε 352 . Φ =4,480, δ . Φ =128 GM), Flu2 ( ε 384 . Φ =2,214, δ . Φ =44 GM) and Flu3 ( ε 441 . Φ =11,333, δ.Φ =192 GM), when compared with the corresponding probes U1 /2/3 ( ε 352 . Φ =~1,000, δ.Φ =17 GM), U4 /5/6 ( ε 384 . Φ =~320, δ.Φ <1 GM) and U7 /8/9 ( ε 441 .Φ =1,680, δ.Φ =29 GM) at their excitation wavelengths, clearly illustrated the anticipated fluorescence ‘Switch-ON’ effect of the probes upon enzymatic release of the propylamine group ( Fig. 1a ). Finally, all probes remained stable in aerated, aqueous buffer for days at room temperature, and Flu1/2/3 showed excellent photostability at their excited wavelengths ( Supplementary Fig. 3d ). Table 1 Photophysical and enzymatic properties of Flu1/U1/U2. Full size table We next assessed the enzymatic activities of U1 –9 with recombinant human MAO-A and MAO-B. Typically, the assays were carried out with each probe (2.0 μM) and the corresponding enzyme (10 μg ml −1 ) in HEPES buffer at 37 °C and the fluorescence was measured over a period of 2 h. The commercially available Amplex Red MAO Assay kit was used as a reference, under similar assay conditions, to normalize the relative MAO-A/B activities. As shown in Fig. 2a (and Supplementary Fig. 4a ), with the Amplex kit, both enzymes produced significant fluorescence increases, with MAO-A consistently exhibiting comparatively higher enzymatic activity than MAO-B (insets). With U1 –9 on the other hand, almost none of the probes (except U2 /3) produced any significant fluorescence increase with MAO-A, even after prolonged incubation, indicating that they were poor substrates of the enzyme. On the contrary, with MAO-B, U1 /2 exhibited significant fluorescence increases, while U3 produced weak but measurable fluorescence increase. These results indicate, and supported by our docking results, that due to the optimized size of the acedan reporter in preferential binding to the longer and narrower ‘substrate’ cavity of MAO-B, U1 /2/3 were indeed MAO-B-specific probes. As was observed previously [17] , [18] , [19] , [20] , tuning the alkylation state of the propylamine group in these probes provided another level of reactivity control to further differentiate MAO-B/A selectivity. U1 was thus taken further for all subsequent experiments due to its ability to register the greatest fluorescence ‘Switch-ON’ response to MAO-B. To further confirm U1 ’s selectivity, the MAO-B/U1 enzymatic assay was repeated in the presence of either CL (a known MAO-A-selective inhibitor with reported A/B IC 50 values of 1.2 nM/630 nM, respectively) [40] or PA (a known MAO-B-selective inhibitor with reported A/B IC 50 values of 4.3 μM/0.14 μM, respectively) [40] . As shown in Fig. 2b , PA caused nearly complete suppression of MAO-B-induced increase in U1 fluorescence, while CL caused only partial suppression of the same fluorescence increase, indicating that this increase was likely originated entirely from MAO-B activity. The partial inhibition of MAO-B activity by CL is not surprising since its residual cross-inhibition against this enzyme is only approximately fourfold less potent than PA (for example, 630 versus 140 nM). Similar results were obtained with MAO-B/Amplex kit (inset). We next carried out detailed kinetic studies of the MAO-B/U1 assay and obtained the corresponding Michaelis–Menten constants ( K m =8.33±0.25 μM, K cat =0.31 min −1 , V max =2.67 nmol mg −1 min −1 ; see Fig. 2c and Table 1 ). As U1 produced insignificant fluorescence increase with MAO-A, even after prolonged incubation and with a large amount of the enzyme, we were unable to obtain its kinetic data with this enzyme. The K m value of U1 was lower than that of the previously reported MAO-B-specific tetrahydropyridine substrate [22] , indicating U1 would serve as a much better MAO-B-specific imaging probe. Concurrently, time-dependent fluorescence measurement was carried out with MAO-B/U1 reactions ( Fig. 2d ), and the results were extrapolated to provide the corresponding reaction constants of k app =3.73±0.12 × 10 4 M −1 min −1 . The expected release of Flu1 was further confirmed using HPLC-MS (inset), showing the direct conversion of U1 to Flu1 with no detectable intermediate formation. We thus concluded that U1 is indeed a two-photon probe suitable for sensitive and continuous reporting of MAO-B activities with minimal cross-reactivity towards MAO-A. 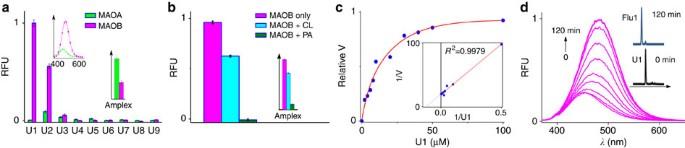Figure 2: Enzymatic properties of MAO-B-specific probeU1. (a) Relative-fluorescence reading ofU1–9 (2.0 μM) upon incubation with 10 μg ml−1MAO-A (green) or MAO-B (purple) for 2 h at 37 °C in HEPES buffers (pH 7.5). Insets: (left) representative excited fluorescence emission spectra of the enzyme/U1 reaction and (right) relative-fluorescence reading of the enzyme/Amplex Red kit at the 2 h time point. (b) Relative-fluorescence reading ofU1(2.0 μM) and recombinant MAO-B (10 μg ml−1) after 2 h at 37 °C, with no inhibitor (purple), 200 μM CL (blue) or 200 μM PA (green). Inset: similar results obtained from the Amplex kit. Error bars ina,brepresent s.e.m.,n=3. (c) Kinetic studies of MAO-B/U1 enzymatic reaction over aU1-concentration range 0–100 μM with 10 μg ml−1MAO-B at 37 °C. Inset: fitted Linewearver–Burk plot. The corresponding kinetic data are summarized inTable 1. (d) Time-dependent fluorescence emission spectra of the reaction between MAO-B (10 μg ml−1) andU1(1.0 μM) over the course of 2 h. Inset: HPLC-MS analysis of the MAO-B/U1 reaction, showing the direct conversion ofU1to Flu1 with no detectable intermediate formation. The HPLC profiles were recorded on a Shimadzu SPD-20A detector (350 nm). Figure 2: Enzymatic properties of MAO-B-specific probe U1 . ( a ) Relative-fluorescence reading of U1 –9 (2.0 μM) upon incubation with 10 μg ml −1 MAO-A (green) or MAO-B (purple) for 2 h at 37 °C in HEPES buffers (pH 7.5). Insets: (left) representative excited fluorescence emission spectra of the enzyme/U1 reaction and (right) relative-fluorescence reading of the enzyme/Amplex Red kit at the 2 h time point. ( b ) Relative-fluorescence reading of U1 (2.0 μM) and recombinant MAO-B (10 μg ml −1 ) after 2 h at 37 °C, with no inhibitor (purple), 200 μM CL (blue) or 200 μM PA (green). Inset: similar results obtained from the Amplex kit. Error bars in a , b represent s.e.m., n =3. ( c ) Kinetic studies of MAO-B/U1 enzymatic reaction over a U1 -concentration range 0–100 μM with 10 μg ml −1 MAO-B at 37 °C. Inset: fitted Linewearver–Burk plot. The corresponding kinetic data are summarized in Table 1 . ( d ) Time-dependent fluorescence emission spectra of the reaction between MAO-B (10 μg ml −1 ) and U1 (1.0 μM) over the course of 2 h. Inset: HPLC-MS analysis of the MAO-B/U1 reaction, showing the direct conversion of U1 to Flu1 with no detectable intermediate formation. The HPLC profiles were recorded on a Shimadzu SPD-20A detector (350 nm). Full size image Imaging of MAO-B-specific activities in live cells/tissues We investigated whether U1 could be used for real-time imaging of MAO-B-specific activities present in mammalian proteome lysates, live cells and deep tissues. Human-derived HepG2 (hepatocellular carcinoma) and SH-SY5Y (neuroblastoma) cells are two well-established disease cell lines possessing elevated levels of MAO-B and MAO-A activities, respectively [41] , [42] , and this was confirmed using western blotting (WB) analysis of the endogenous protein expression levels with the corresponding cell lysates (inset in Fig. 3a ). We further confirmed the presence of MAO-B, but not MAO-A, activities in HepG2 cell lysates by directly incubating them with U1 , with and without CL and PA ( Fig. 3a and Supplementary Figs 6 and 7 ); results showed that these lysates produced significant PA-sensitive fluorescence signals. U1 -treated SH-SY5Y cell lysates, on the other hand, failed to generate any above-background fluorescence under all tested conditions, which further supports the extremely high selectivity of U1 in detecting MAO-B activities even in complex proteomes. Unlike general MAO-detecting assays such as the Amplex kit or other antibody-based enzyme-linked immunosorbent assay (ELISA) assays, all of which require the physical isolation of MAO-B protein, U1 provides a simple and rapid means to selectively report, in real-time, endogenous MAO-B activities in crude proteomes. In fact, fluorescence measurements of U1 -treated proteome lysates obtained from eight different mammalian cell lines (HEK293, PC-3, CNE-1, HeLa, HCT116, A549, MCF7 and HepG2) provided a good correlation between the fluorescence read-outs and their endogenous MAO-B expression levels measured from the corresponding WB experiments ( Supplementary Fig. 8 ). This is a useful feature that may be explored in future for in situ screening of potential MAO-B inhibitors [43] . 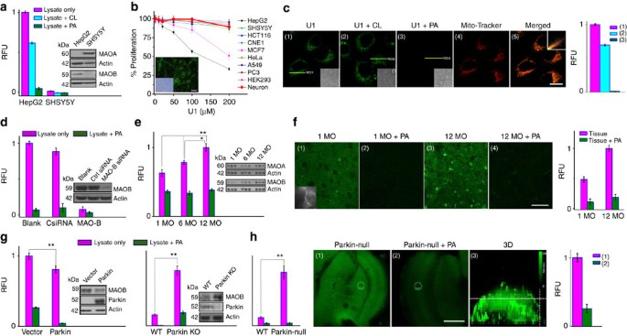Figure 3: Fluorescence detection and bioimaging of MAO-B activities byU1in live mammalian cells/tissues and parkin-related PD models. (a) Relative-fluorescence reading ofU1(2.0 μM)+lysates of HepG2/SH-SY5Y cells, with no inhibitor (purple), CL (blue) or PA (green). Inset: WB results. (b) The cytotoxicity ofU1against mammalian cell lines and mouse primary neurons (red line). Inset: immunofluorescence/bright field images of purified cortical neurons from the cortex of E17.5 mouse. Scale bar=50 μm. (c) Left: one-photon image of HepG2 cells with (1)U1(10 μM), (2)U1/CL, (3)U1/PA, (4) Mito-Tracker and (5) Merged-image of (1)/(4) with colocalization analysis (inset;R=0.82).λex=405 nm. Scale bar=10 μm. Inset: differential interference contrast images. Right: graphical quantification of average fluorescence intensity of HepG2 image panels 1–3 at the indicated position. (d) Relative-fluorescence reading ofU1(2.0 μM)+lysates of siRNA knockdown HepG2 cells using MAO-B-targeting siRNA (MAO-B) and non-targeting control siRNA (CsiRNA), with/without PA (green/purple). Inset: WB results. (e) Relative-fluorescence reading ofU1(2.0 μM)+brain lysates of 1/6/12-month-old (1/6/12-MO) mice, with/without PA (green/purple). Inset: WB results. (f) Left: two-photon image of the SNpc region of fresh 1/12-MO-mouse brain slices with (1)/(3)U1(100 μM), (2)/(4)U1(100 μM)+PA. 120 μm depth with × 40 magnification atλex=780 nm. Scale bar=50 μm. Right: average fluorescence intensity profiles of mouse brain image panels (1)/(2)/(3)/(4). (g) Left: relative-fluorescence reading ofU1(2.0 μM)+lysates of parkin-transfected HepG2 cells. Inset: WB results. Right: relative-fluorescence reading ofU1(2.0 μM)+lysates of WT and parkin-knockout embryonic fibroblasts. Inset: WB results. (h) Left: relative-fluorescence reading ofU1(2.0 μM)+total lysates of WT and 20-day-old parkin-null-femaleDrosophila. Middle: two-photon image of fresh brain slices of 20-day-old parkin-nullDrosophilawith (1)U1(100 μM) andU1(100 μM)+PA (200 μM). Depth (100 μm) with × 40 magnification atλex=780 nm. Parkin-null image panel (3) is a reconstructed 3D two-photon image of (1). Scale bar=150 μm. Right: average fluorescence intensity profiles of parkin-null image panels (1)/(2) at the position indicated. *P<0.05, **P<0.01,n=3, Student’st-test, two-tailed ine,g,h; error bars ina,c–hrepresent s.e.m. Full-size WB can be found inSupplementary Fig. 15. Figure 3: Fluorescence detection and bioimaging of MAO-B activities by U1 in live mammalian cells/tissues and parkin-related PD models. ( a ) Relative-fluorescence reading of U1 (2.0 μM)+lysates of HepG2/SH-SY5Y cells, with no inhibitor (purple), CL (blue) or PA (green). Inset: WB results. ( b ) The cytotoxicity of U1 against mammalian cell lines and mouse primary neurons (red line). Inset: immunofluorescence/bright field images of purified cortical neurons from the cortex of E17.5 mouse. Scale bar=50 μm. ( c ) Left: one-photon image of HepG2 cells with (1) U1 (10 μM), (2) U1 /CL, (3) U1 /PA, (4) Mito-Tracker and (5) Merged-image of (1)/(4) with colocalization analysis (inset; R =0.82). λ ex =405 nm. Scale bar=10 μm. Inset: differential interference contrast images. Right: graphical quantification of average fluorescence intensity of HepG2 image panels 1–3 at the indicated position. ( d ) Relative-fluorescence reading of U1 (2.0 μM)+lysates of siRNA knockdown HepG2 cells using MAO-B-targeting siRNA (MAO-B) and non-targeting control siRNA (CsiRNA), with/without PA (green/purple). Inset: WB results. ( e ) Relative-fluorescence reading of U1 (2.0 μM)+brain lysates of 1/6/12-month-old (1/6/12-MO) mice, with/without PA (green/purple). Inset: WB results. ( f ) Left: two-photon image of the SNpc region of fresh 1/12-MO-mouse brain slices with (1)/(3) U1 (100 μM), (2)/(4) U1 (100 μM)+PA. 120 μm depth with × 40 magnification at λ ex =780 nm. Scale bar=50 μm. Right: average fluorescence intensity profiles of mouse brain image panels (1)/(2)/(3)/(4). ( g ) Left: relative-fluorescence reading of U1 (2.0 μM)+lysates of parkin-transfected HepG2 cells. Inset: WB results. Right: relative-fluorescence reading of U1 (2.0 μM)+lysates of WT and parkin-knockout embryonic fibroblasts. Inset: WB results. ( h ) Left: relative-fluorescence reading of U1 (2.0 μM)+total lysates of WT and 20-day-old parkin-null-female Drosophila . Middle: two-photon image of fresh brain slices of 20-day-old parkin-null Drosophila with (1) U1 (100 μM) and U1 (100 μM)+PA (200 μM). Depth (100 μm) with × 40 magnification at λ ex =780 nm. Parkin-null image panel (3) is a reconstructed 3D two-photon image of (1). Scale bar=150 μm. Right: average fluorescence intensity profiles of parkin-null image panels (1)/(2) at the position indicated. * P <0.05, ** P <0.01, n =3, Student’s t -test, two-tailed in e , g , h ; error bars in a , c – h represent s.e.m. Full-size WB can be found in Supplementary Fig. 15 . Full size image To investigate the capability of U1 for real-time bioimaging of MAO-B activities in live cells, we used two complementary techniques—that is, flow cytometry and confocal microscopy. We first established that U1 was minimally cytotoxic to most mammalian cells and primary neurons at concentrations up to 50 μM ( Fig. 3b ). Flow cytometry experiments with U1 -treated HepG2 cells revealed a marked increase in the population of highly fluorescent cells, a phenomenon that was suppressed by PA treatment ( Supplementary Fig. 10 ). In parallel, real-time imaging of U1 -treated live HepG2 cells with confocal microscopy demonstrated a progressive increase in fluorescence, detectable only inside the mitochondria of the cells ( Fig. 3c and Supplementary Figs 11,12 and Supplementary Video 1 ). This fluorescence was completely suppressed by PA but not by CL. Subcellular fractionation experiments independently verified that endogenous MAO-B expression was, as previously reported [1] , [7] , [20] , predominantly localized to mitochondria of HepG2 cells ( Supplementary Fig. 9a ). On the other hand, despite its potentially positively charged amine head group under physiological conditions, U1 was shown to be present in both the cytosol and mitochondria of U1 -treated HepG2 cells ( Supplementary Fig. 9b ). We further tested proteome lysates obtained from siRNA experiments, in which endogenous MAO-B expression in HepG2 cells was knocked down ( Fig. 3d ); results showed that, in the absence of MAO-B expression, U1 -treated HepG2 cells failed to generate any above-background fluorescence readings. We thus conclude that U1 is a cell-permeable, non-toxic small molecule probe capable of highly sensitive imaging of MAO-B activities in live mammalian cells with good spatial resolution. Encouraged by these results, we next determined whether U1 could be used to image MAO-B activities in deep tissues such as mouse brains using two-photon microscopy (TPM), and report age-associated increases in MAO-B expression. We first took brain lysates isolated from C57/B6 mice of different ages (that is, 1, 6 and 12 months) and treated them (300 μg ml −1 ) with U1 for 2 h ( Fig. 3e ); consistent with previous reports [2] , [7] , we found an age-dependent increase in U1 fluorescence readings caused by MAO-B activities, which were further confirmed by PA treatment ( Fig 3e , P <0.01, n =3, Student’s t -test, two-tailed, error bars represent s.e.m.). This result was further supported by the corresponding WB analysis that revealed an increase in MAO-B but not MAO-A expression with age (inset). To directly image MAO-B activities using TPM, sections of the same mouse brains (1- and 12-month-old) were treated with U1 , with and without PA treatment ( Fig. 3f ); with the ability of TPM to directly image the SNpc at 120-μm depth, we were able to exclusively focus on this region of the mouse brain where high levels of MAO-B-expressing astrocytes were populated (hence most relevant to PD imaging/diagnosis). Supporting our results above, these TPM images revealed higher PA-sensitive fluorescence increases in the SNpc of 12-month-old mice, the fluorescence intensity profiles of which were further graphically quantified (inset). Imaging parkin-related PD models in vitro / in vivo by using U1 With this newly discovered MAO-B-specific imaging probe (for example, U1 ), we next investigated its potential applications for evaluation of the relationship between MAO-B expression and dopaminergic neuronal homoeostasis in PD models. Parkin is a component of a multiprotein E3 ubiquitin ligase complex in the ubiquitin–proteasome system that mediates protein degradation [44] . Previously, the loss of parkin function associated with recessive parkinsonism was reported to promote the expression of MAO-B, which is thought to contribute towards the pathogenicity in parkin-related PD cases [45] . To examine whether U1 could faithfully report the inverse relationship between parkin and MAO-B expression, proteome lysates prepared from HepG2 cells transfected with a parkin-expressing gene were treated with U1 , with and without PA treatment ( Fig. 3g left); consistent with the reported role that increase in parkin expression suppresses MAO-B expression (inset) [45] , we observed a significant reduction in PA-sensitive U1 fluorescence from parkin-transfected cells versus vector-transfected control cells ( P <0.01, n =3, Student’s t -test, two-tailed). The reverse scenario was also observed in U1 -treated proteome lysates prepared from mouse embryonic fibroblasts derived from parkin-knockout mice ( Fig. 3g right); both PA-sensitive U1 fluorescence and the corresponding MAO-B expression (determined by WB) were significantly higher in parkin-knockout mouse embryonic fibroblasts ( Fig. 3g right, P <0.01, n =3, Student’s t -test, two-tailed, error bars represent s.e.m.). Although parkin-deficient mice generally fail to show robust signs of parkinsonism, we and others had demonstrated that Drosophila parkin-null mutants exhibit features that mirror the human PD patients, including dopaminergic neurodegeneration and concomitant locomotion defects [28] . We therefore investigated whether U1 could be used to examine the relationship between parkin and MAO-B in vivo using this insect PD model. Proteome lysates from 20-day-old wild-type (WT) and parkin-null flies were prepared and tested with U1 . Similarly, we also carried out TPM imaging with U1 -treated dissected brains of these flies at a depth of 100 μm ( Fig. 3h and Supplementary Fig. 13 ); in good agreement with above cell-based results, both the lysate and the TPM experiments indicate significantly higher PA-sensitive U1 fluorescence readings from parkin-null flies compared with the WT flies ( P <0.01, n =3, Student’s t -test, two-tailed, error bars represent s.e.m.). Owing to the lack of suitable antibodies to detect Drosophila MAO-B, we were unable to unequivocally establish the expression level of this protein in these parkin-null flies by WB analysis; our PA-treated samples, however, suggest that these U1 fluorescence signals likely originated exclusively from MAO-B. A reconstructed, two-photon fluorescence three-dimensional (3D) image of parkin-null Drosophila brain was generated (parkin-null image in Fig. 3h and Supplementary Video 2 ), to further demonstrate the capability of U1 for high-resolution, real-time imaging of MAO-B activities in the whole brain of small insect/animal PD models. Detecting MAO-B activities in PD patients’ samples Having demonstrated the ability of U1 for highly specific detection of MAO-B activities from various biological sources (mammalian cells, flies and mice), some of which were derived from parkin-derived PD models, we were keen to assess whether U1 could be used with clinically relevant samples by providing a convenient means for rapid and sensitive detection of elevated levels of MAO-B activities, which are a hallmark of PD patients. Proteome lysates prepared from B lymphocytes derived from local PD patients, as well their corresponding age-matched controls, were treated with U1 , and fluorescence signals obtained from the PA-sensitive MAO-B-specific activities were measured. Notably, only MAO-B is known to be expressed in B lymphocytes [46] . As shown in Fig. 4a , in all three PD patient samples, significantly higher U1 fluorescence was detected when compared with control normal samples ( P <0.001, n =3, Student’s t -test, two-tailed, error bars represent s.e.m. ), indicative of an obvious increase in MAO-B expression in the lymphocytes of these PD patients (a conclusion further validated by WB analysis; see inset in Fig. 4a ). As controls, we also carried out similar experiments with lysates prepared from fibroblasts of the same patients, whose MAO-B expression levels were comparable to those of control patients as determined using WB analysis ( Fig. 4b inset); results showed nearly equal U1 fluorescence readings from all samples. Similar results were also obtained from the imaging-based experiments by using one- and TPM, which again showed exclusive mitochondria-localized, MAO-B activities in the PD patient’s fibroblast cells ( Supplementary Fig. 14 ). We thus concluded that the difference in MAO-B activity profiles between control and PD patients are cell-type-specific. This finding is important as it suggests that the activity of MAO-B in peripheral blood cells may potentially be used as a convenient surrogate biochemical marker for PD diagnosis, and perhaps even as a preclinical marker for at-risk individuals who are otherwise asymptomatic. At present, there is no reliable biomarker for PD, either at the diseased or at the preclinical stage (except for DA-based PET imaging, which is costly and requires highly specialized skills to perform [47] ) [48] . We thus propose that MAO-B might render itself as a useful and economical biomarker for PD. Pending proper future evaluations of the status of MAO-B by using U1 in a large cohort of case–control population, we are keen to develop this probe further into a commercial test kit for PD diagnostics. 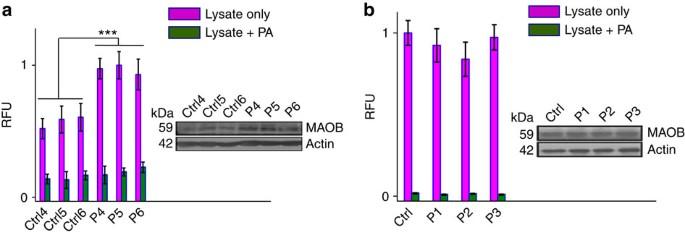Figure 4: U1-assisted detection of MAO-B for potential clinical diagnostics of PD in human. (a) Relative-fluorescence reading ofU1(2.0 μM) after incubation with 500 μg ml−1proteome lysates of human B lymphocytes obtained from (P4–6) PD patients and (Ctrl4–6) aged-matched normal controls. Inset: WB results of the corresponding samples. (b) Relative-fluorescence reading ofU1(2.0 μM) after incubation with 300 μg ml−1lysates prepared from fibroblasts of PD patients (P1–3) and the corresponding age-matched controls (Ctrl). ***P<0.001,n=3, Student’st-test, two-tailed ina; error bars ina,brepresent s.e.m. Inset: WB results of the corresponding samples. All enzymatic assays were carried out at 37 °C in HEPES buffers (pH 7.5) for 2 h. Inhibition assays were performed by PA treatment (200 μM) before the addition ofU1. Full-size western blots can be found inSupplementary Fig. 15. Figure 4: U1-assisted detection of MAO-B for potential clinical diagnostics of PD in human. ( a ) Relative-fluorescence reading of U1 (2.0 μM) after incubation with 500 μg ml −1 proteome lysates of human B lymphocytes obtained from (P4–6) PD patients and (Ctrl4–6) aged-matched normal controls. Inset: WB results of the corresponding samples. ( b ) Relative-fluorescence reading of U1 (2.0 μM) after incubation with 300 μg ml −1 lysates prepared from fibroblasts of PD patients (P1–3) and the corresponding age-matched controls (Ctrl). *** P <0.001, n =3, Student’s t -test, two-tailed in a ; error bars in a , b represent s.e.m. Inset: WB results of the corresponding samples. All enzymatic assays were carried out at 37 °C in HEPES buffers (pH 7.5) for 2 h. Inhibition assays were performed by PA treatment (200 μM) before the addition of U1 . Full-size western blots can be found in Supplementary Fig. 15 . Full size image As the predominant isoform of MAOs found in the human brain, the unusually high MAO-B activity observed in the brain is directly responsible for a number of neurodegenerative diseases including PD [2] , [8] . PD is a degenerative disorder in the central nervous system, resulting from the death of DA-generating cells in the SNpc of the patient’s midbrain. At present, there is no reliable diagnostic biomarker for PD, either at the diseased or at the preclinical stage. Consequently, PD patients are mainly diagnosed based on symptoms, with neuroimaging tests such as the DA-based PET imaging being used for confirmation, although its high cost precludes its routine use in the clinic [47] . No cure for PD is presently available; however, several MAO-B inhibitors have been shown to provide relief from the symptoms and are currently being used for the treatment of early-stage PD [11] , [12] , [13] . The biological and clinical importance of MAO-B in PD has led us to successfully develop U1 , a first-generation, two-photon fluorogenic imaging probe. The extremely high MAO-B selectivity observed by U1 was unequivocally established under a variety of experimental conditions, both in vitro and in situ , with recombinant enzymes or with MAO-B-expressing crude proteomes. We show that the probe may be used for in situ screening of potential MAO-B inhibitors [43] . We further show that U1 could be used for real-time measurements of endogenous MAO-B activities across various established PD models and clinically relevant specimens. Mutations in the parkin gene are known to cause a familial form of PD, with recessive parkinsonism and promotion of MAO-B expression, leading to dopaminergic cell death [47] . However, how this process occurs remains unclear. With U1 , we showed, for the first time, that two-photon fluorescence microscopy could be carried out directly for sensitive and high-resolution imaging of MAO-B-specific activities in deep tissues such as brains of age-associated mice and parkin-null Drosophila . The lack of a good genetic mouse model of parkin-related PD has thus far precluded our further investigation in a mammalian species, but previously published results with the parkin-null Drosophila mutants used in the current study clearly demonstrate that these fly models exhibit characteristic PD symptoms including dopaminergic neurodegeneration and concomitant locomotion defects and are therefore suitable models for PD research [28] . Together with U1 , this system may be used in future to unlock the molecular basis behind the inverse relation of parkin and MAO-B at the organism level. Notably, U1 has no apparent toxicity in most mammalian cells and mouse primary neurons at concentrations that are useful for most practical purposes, thus providing the opportunity to monitor MAO-B activities in small animals over various stages of disease development. Finally, U1 -assisted fluorescence detection of MAO-B activities in clinical samples obtained from PD patients further emphasizes the potential diagnostic values of this probe for this disease. Our finding that elevated MAO-B activities are present only in human B lymphocytes, but not in fibroblasts, of PD patients provides clues that MAO-B in peripheral blood cells of a patient might serve as a useful and economical biomarker for rapid detection of this disease. Much more work will, however, need to be carried out to further substantiate this preliminary finding. Taken together, the discovery of U1 , a two-photon small molecule probe suitable for specific and sensitive detection of MAO-B activities in a variety of biological systems including established PD models, is important in the research of PD. Our results provide important starting points for using small molecule imaging techniques to explore the chemistry and biology of MAO-B at the organism level and should provide useful tools for basic research, diagnosis and drug discovery in the combat against PD. Chemical synthesis Briefly, the methylamine group in Flu1 was activated as a carbamic chloride (for example, compound 4 ), which was subsequently reacted with t -Boc-protected primary or secondary propylamine under basic conditions (to afford compounds 7/8 ) followed by deprotection with trifluoroacetic acid to give U1/2 . Compound 4 was directly coupled with 3-dimethylamino-1-propanol to afford U3 . The original 1 H- and 13 C-NMR spectra are available in Supplementary Figs 16–57 . 3-Aminopropyl(6-acetylnaphthalen-2-yl)(methyl)carbamate (U1) Compound 7 (70 mg, 0.18 mmol) was dissolved in a cold (0 °C) solution of 1:1 trifluoroacetic acid and CH 2 Cl 2 (5 ml). The solution was kept in the dark and stirred for 1 h at 0 °C before being allowed to warm to room temperature and stirred for an additional 2 h. The solvents were removed in vacuo, and the residue was dissolved in DMSO, filtered and purified to homogeneity by a Semi-Prep HPLC on a C 18 column. After lyophilization, U1 was isolated as a pink powder (31 mg, 59% yield). 1 H NMR (300 MHz, CDCl 3 ) δ 1.92 (bs, 2H), 2.67 (s, 3H), 2.92 (bs, 2H), 3.33 (s, 3H), 4.15 (t, J =5.7 Hz, 2H), 7.42 (d, J =10.2 Hz, 1H), 7.64 (s, 1H), 7.79 (d, J =8.7 Hz, 1H), 7.90 (d, J =9.0 Hz, 1H), 7.98 (d, J =10.2 Hz, 1H), 8.38 (s, 1H); 13 C NMR (75 MHz, CDCl 3 ) δ 26.60, 36.58, 37.66, 40.68, 62.22, 122.92, 124.60, 125.39, 128.15, 129.73, 130.38, 130.62, 134.61, 135.71, 142.62, 155.76, 198.06. IT-TOF-MS: m/z [M+H] + calcd: 301.15, found: 301.11. Molecular modelling To compare the active-site cavities of MAO-A and -B, the crystallographic structures of CL/MAO-A (PDB code: 2BXR) and PA/MAO-B (PDB code: 1GOS) were retrieved from the PDB, and the surface of active-site cavities shown in ‘chicken-wire’ was displayed using PyMol (version 0.99, DeLano Scientific LLC). To demonstrate the specific recognition of U1 with respect to MAO-B compared with MAO-A, docking was carried out using the Autodock Vina software (version 1.56, The Scripps Research Institute) [49] , [50] . For substrate docking with protein, the crystallographic structures of MAO-A (PDB code: 2Z5X) and MAO-B (PDB code: 2BK3) were retrieved from the PDB. Explicit hydrogen atoms were added, and all water molecules were then deleted. The ligand was removed, and the protein structure was processed using AutoDock Tools as setting Grid box size of 40/40/40 around centre 22.073/128.241/16.19 and 42/52/46 around centre 36.739/31.292/-12.149 for MAO-A and -B, respectively. Probes U1/4/7 and tyramine were prepared for docking by using AutoDock Tools to assign AD4 atom types, calculate Gasteiger charges and set all rotatable bonds as active torsions. The ligand was docked into the protein using AutoDock Vina. The exhaustiveness parameter was set as default. Not only the macromolecule molecular solid-ligand site structures were displayed by PyMol, but also a directly distance measurement was carry out between C5 of FAD and terminal N atom of ligands to identify recognition potency ( Supplementary Figs 1 and 2 ). Enzymatic assays All enzymatic assays were carried out in HEPES buffer (pH 7.5) supplemented with 0.1% Triton X-100 at 37 °C. Activities of recombinant MAO-A and MAO-B proteins were normalized with the Amplex Red kit (A12214) by using p -tyramine hydrochloride as substrate. The activity was assayed spectrophotometrically by monitoring the rate of resorufin formation at 560 nm following the manufacturer’s guidelines. All measurements were performed in triplicate. Proteome lysates from cells or tissues were prepared similarly as those for WB analysis. Next, enzymatic assays were performed in a final volume to 200 μl (final concentration: 10, 300 and 500 μg ml −1 for purified proteins, lysates and B lymphocytes, respectively) and 2.0 μM of the probe (for example, U1 ). For inhibition assays, either CL or PA (200 μM) was pre-incubated with the biological samples for 2 h before the addition of U1 (2.0 μM) for another 2–3 h. The fluorescence was monitored at 470 nm ( λ ex =350 nm). For kinetic studies, U1 (concentration ranged from 0 to 100 μM) was added to a solution of MAO-B (final concentration: 10 μg ml −1 ). Time-dependent enzymatic reaction of U1 /MAO-B was closely monitored spectrofluorometrically and using HPLC-MS. The reaction constant was defined from the half-life equation for a second-order reaction dependent on one second-order reactant ( k = t 1/2 −1 [A] 0 −1 ). All fluorometric measurements were performed on a Perkin-Elmer LS50 spectrofluorometer. Drosophila , mouse brain tissue and clinical samples of PD patients’ culture The parkin-null mutant Drosophila was a kind gift from J. Chung and K.S. Cho (Korea Advanced Institute of Science and Technology, Daejeon, Korea). All flies were grown on corn meal–molasses medium and maintained at 25 °C. Protein extracts for fluorescence assay were prepared by homogenizing 10 fly heads and thoraces in lysis buffer (phosphate-buffered saline (PBS) with 1% SDS, Phenylmethylsulfonyl Fluoride, Aprotinin) with glass homogenizer and then sonicated with Sonics (VCX 130). The siRNA knockdown experiment was conducted following protocols provided by the vendor (Thermal Scientific). Briefly, HepG2 cells were seeded in six-well plates and incubated overnight at 37 °C with 5% CO 2 . MAO-B targeting as well as non-targeting siRNA (CsiRNA) and DharmaFECT transfection reagent were diluted in serum-free medium, respectively, and incubated at room temperature for 5 min. The diluted siRNA and transfection reagent were mixed and incubated at room temperature for 20 min. The normal medium of HepG2 cells was removed and replaced with antibiotic-free medium with mixtures of siRNA and transfection reagent. The final concentration of siRNA was 12.5 nM. After being incubated for 48 h, the cells were collected, lysed and tested for MAO-B expression (with anti-MAO-B WB) and enzymatic activity (with U1 ). All procedures involving animals were approved by and conformed to the guidelines of our Institutional Animal Care and Use Committee at the National Neuroscience Institute. One/six/twelve-month-old male c57 mice were killed with cervical dislocation. To prepare lysates, the brain was first homogenized in lysis buffer (PBS with 1% triton X-100, Phenylmethylsulfonyl Fluoride, Aprotinin) with glass homogenizer and then sonicated with Sonics (VCX 130). The PD patient’s fibroblasts were purchased from Coriell Cell Repositories. The ID of the patients’ derived cell lines were AG08395, AG04148 and AG20439, respectively. Control fibroblasts were purchased from GIBCO (Cat No: C-013-5C). The fibroblasts were cultured in the medium (DMEM with 10% fetal bovine serum, 1% Pen-Strep, 2 mM glutamine, 0.1% beta -Mercaptoethanol, non-essential amino acids) in a humidified 5% CO 2 incubator at 37 °C. Cells were grown to 80~90% confluency. Then, fibroblasts were washed with cold PBS and lysed in lysis buffer (PBS with 1% triton X-100, Phenylmethylsulfonyl Fluoride, Aprotinin). The B lymphocytes were ordered from Coreil Cell Repositories (New Jersey, USA), including three strains (ND00038, ND00287 and ND02509) derived from sporadic PD patients and three strains (ND01504, ND01929 and ND02296) from age-matched healthy controls. The B lymphocytes were cultured, in suspension, in RPMI 1640 with 2 mM L-glutamine, 15% fetal bovine serum, 1% penicillin/streptomycin in 37 °C incubator with 5% CO 2 . When the cells reached one million viable cells per ml, they were splitted. To prepare cell lysates, cells were centrifuged and the cell pellets were washed with cold PBS and then lysed in lysis buffer (PBS with 1% SDS, Phenylmethylsulfonyl Fluoride, Aprotinin). Soluble fractions of all types of lysates were separated with centrifugation at 13,500 r.p.m. at 4 °C for 15 min. General procedures for two-photon deep-tissue imaging Tissues used in our imaging experiments were fresh brains of 20-day-old live female Drosophila and 1/12-month-old mice. For mice, brains were surgically removed from the mouse head and immediately transferred into ice-artificial cerebrospinal fluid (ACSF; 138.6 mM NaCl, 3.5 mM KCl, 21 mM NaHCO 3 , 0.6 mM NaH 2 PO 4 , 10 mM D-glucose, 1 mM CaCl 2 and 3 mM MgCl 2 ). Coronal slices, which contain Substantia nigra, were cut into 200-μm-thick sections using a vibrating blade microtome in ACSF. Slices were incubated with 100 μM U1 in ACSF bubbled with 5:95 (v/v) of CO 2 /O 2 at 37 °C for 2 h. For inhibition experiments, the brains were treated with PA (200 μM) 2 h before incubation with U1 . Treated brains were then transferred to poly-L-lysine-coated coverslips. The images were taken at 120-μm depth by changing the z axis thickness. For Drosophila , whole brains were prepared from a series of 20-day-old WT and parkin-null Drosophila . Brains were incubated with U1 (3 h) in DMEM under a humidified atmosphere of 5:95 (v/v) of CO 2 /air at 37 °C. For inhibition experiments, brains were treated with PA (200 μM) 2 h before incubation with U1 . Treated brains were subsequently transferred to poly-L-lysine-coated coverslips. The images were taken at 100-μm depth by changing the z axis thickness. 3D TPM images (parkin-null image Fig. 3h and Supplementary Video 2 ) of parkin-null Drosophila whole brains were taken from top to bottom along the z axis of the brains, and reconstructed with Leica Application Suite Advanced Fluorescence. Statistical analysis All data are expressed as means±s.e.m. The data were accumulated under each condition from at least three independent experiments. The statistical analyses were performed using the Student’s t -test. Other methods Additional experimental information and results (chemistry and biology) are provided in Supplementary Methods . Note: Supplementary information is available on the Nature Communications website. How to cite this article: Li, L. et al . A sensitive two-photon probe to selectively detect monoamine oxidase B activity in Parkinson’s disease models. Nat. Commun. 5:3276 doi: 10.1038/ncomms4276 (2014).